Rapid adaptation to food availability by a dopamine-mediated morphogenetic response Food can act as a powerful stimulus, eliciting metabolic, behavioural and developmental responses. These phenotypic changes can alter ecological and evolutionary processes; yet, the molecular mechanisms underlying many plastic phenotypic responses remain unknown. Here we show that dopamine signalling through a type-D 2 receptor mediates developmental plasticity by regulating arm length in pre-feeding sea urchin larvae in response to food availability. Although prey-induced traits are often thought to improve food acquisition, the mechanism underlying this plastic response acts to reduce feeding structure size and subsequent feeding rate. Consequently, the developmental programme and/or maternal provisioning predetermine the maximum possible feeding rate, and food-induced dopamine signalling reduces food acquisition potential during periods of abundant resources to preserve maternal energetic reserves. Sea urchin larvae may have co-opted the widespread use of food-induced dopamine signalling from behavioural responses to instead alter their development. Predator–prey interactions can produce developmental and morphological responses with significant ecological and evolutionary implications [1] , [2] , [3] , [4] , [5] . Predator-induced defenses reduce the prey's risk of consumption, whereas prey-induced offenses improve consumption or competitive ability in the predators [1] , [2] , [3] , [6] , [7] , [8] . These phenotypic changes can thus affect trophic interactions, predator and prey population dynamics, community dynamics, and can drive speciation [1] , [2] , [6] . A mechanistic understanding of these responses is necessary to understand their evolution, limitations, adaptive value, and functional consequences [4] , [9] , [10] , but this has remained elusive for prey-induced offenses and all but a few models of predator-induced defenses [11] , [12] . Echinoid larvae exhibit phenotypic plasticity in feeding structure size after feeding is initiated [13] , [14] and also in advance of feeding [15] , providing a tractable developmental model to investigate prey-induced phenotypic plasticity. When food is plentiful, larvae develop smaller feeding arms, whereas when food is scarce, they develop longer feeding arms. Like many other prey-induced responses [6] , [7] , the sea urchin larval response has been described as an offensive response, developing a larger feeding structure when food is scarce in order to improve food acquisition [15] . Such a response, if adaptive, would allow larvae to adjust to the inherent spatial and temporal variability in the supply of their food (algae). It might also allow them to buffer trophic mismatches due to climate change [16] , [17] , as the seasonal peak abundance of some echinoderm larvae in the water column has shifted forward in time [16] . However, the adaptive value and offensive nature of this prey-induced phenotypic response has not been established. Sea urchin larvae may be able to induce the development of longer arms when food is scarce, the assumed offensive response; alternatively, larvae may only be able to inhibit development from a pre-determined maximum to make shorter arms when food is abundant. The alternative hypotheses result in the same observed phenotypes but through different directional mechanisms with very different organismal (offensive versus protective/defensive) and ecological (increasing versus decreasing grazing/predation pressure) consequences and thus different limitations and implications for selection and evolution. In order to distinguish whether long arms are induced in low food density or, conversely, whether short arms are induced at high food density, it is necessary to determine the underlying food-response mechanism. In pre-feeding Strongylocentrotus purpuratus larvae, this developmental response occurs over only a few days and requires direct chemosensation of algae [15] ; thus it is likely to occur through a neurosensory mechanism. We report that dopamine is the neuro-signaling pathway by which algal sensation alters development. Dopamine signalling promotes shortening of larval arm length from a developmentally determined maximum. Thus, unexpectedly, this prey-induced plasticity is not an offensive response to improve resource acquisition. By experimentally manipulating dopamine signalling and arm length, we assess the costs, benefits, and limitations of this phenotypic response and provide evidence to suggest that sea urchin larvae may have co-opted a widely used signalling pathway of food intake for developmental responses. Algae-induced dopamine signalling inhibits arm elongation By screening pharmaceuticals targeted to known sea urchin neurotransmitters, we discovered that dopamine signalling is involved in regulating post-oral arm growth in pre-feeding larvae. We used the length of the skeletal elements in the post-oral arms as a proxy for the size of the feeding apparatus ( Fig. 1a,b ), as this skeletal structure supports the ciliary band with which the larvae capture food particles. As in previous studies [15] , the response to food was manifested as plasticity in post-oral arm length ( Fig. 1c ) rather than global changes in body size ( Fig. 1d ). Thus, body rod length was used here as a control for whole-embryo or nonspecific responses to perturbations, such as sickness. Pharmacological activation of dopamine type-D 2 receptor (DRD2) function with the agonist, quinpirole, inhibited arm elongation, recapitulating the phenotype observed in larvae reared in the presence of abundant food. Post-oral arm length decreased preferentially compared with body rod length with increasing dosage of quinpirole ( Fig. 2a ) providing evidence that the direction of the response may be to inhibit growth of the feeding arms. Furthermore, the short-arm phenotypic response to food was suppressed by antagonizing DRD2 with amisulpride ( Fig. 2b ; Supplementary Table S1 ), suggesting that dopamine functions downstream of algal sensation. 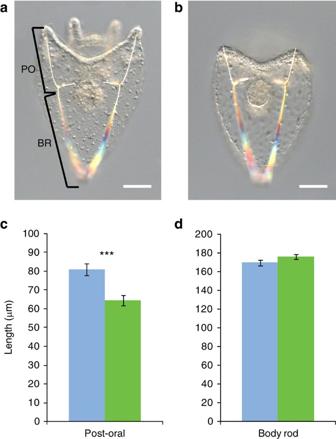Figure 1: Larvae alter the length of their post-oral arms in response to food. Differential interference contrast images of larvae at the end of the pre-feeding period, day 5, cultured without (a) and with (b) algae starting at gastrula stage. The lengths of the post-oral and body rod skeletal elements are indicated by the black lines. Quantification of (c) post-oral arm length, representing a 20.2% (±3.9 s.e.m.) change, and (d) body rod length, representing a 3.9% (±1.5 s.e.m.) change for larvae cultured with (green,n=20) and without (blue,n=18) algae. Student's two-tailedt-test, ***P<0.001. Error bars±s.e.m. BR, body rod; PO, post-oral arm. Scale bars, 50 μm. Figure 1: Larvae alter the length of their post-oral arms in response to food. Differential interference contrast images of larvae at the end of the pre-feeding period, day 5, cultured without ( a ) and with ( b ) algae starting at gastrula stage. The lengths of the post-oral and body rod skeletal elements are indicated by the black lines. Quantification of ( c ) post-oral arm length, representing a 20.2% (±3.9 s.e.m.) change, and ( d ) body rod length, representing a 3.9% (±1.5 s.e.m.) change for larvae cultured with (green, n =20) and without (blue, n =18) algae. Student's two-tailed t -test, *** P <0.001. Error bars±s.e.m. BR, body rod; PO, post-oral arm. Scale bars, 50 μm. 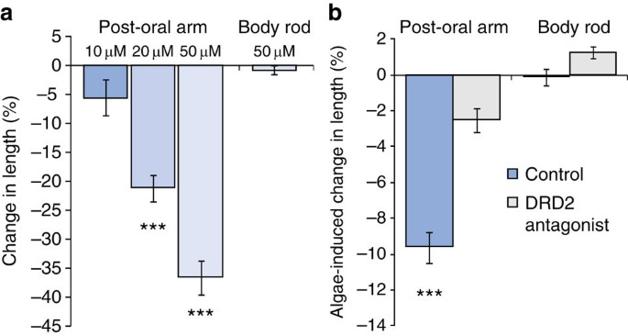Figure 2: Dopamine signalling through type-D2receptors mediates inhibition of skeletal growth by algal sensation. (a) Change in post-oral arm and body rod length for 5-day larvae treated with DRD2 agonist, quinpirole, at the indicated concentrations versus control. One-way ANOVA for post-oral arm length,F3,463=30.586,P<0.0001. Bonferroni-corrected comparisons versus control; ***P<0.001. The decrease in arm length was not due to a global response or sick embryos as body rod length and other aspects of larval morphology did not change with treatment. (b) Change in post-oral arm and body rod length for 5-day larvae cultured with versus without algae for control (blue) and DRD2 antagonist amisulpride, 25 μM, (light grey) treatments. ANOVA (Supplementary Table S1), treatment×algae for post-oral arms,F1,363=7.005,P=0.008 and for body rods,F1,345=1.584,P=0.209; Bonferroni-corrected comparisons without versus with algae (i.e. algae-induced change), ***P<0.001. Error bars±s.e.m. DRD2, dopamine receptor type-D2. Full size image Figure 2: Dopamine signalling through type-D 2 receptors mediates inhibition of skeletal growth by algal sensation. ( a ) Change in post-oral arm and body rod length for 5-day larvae treated with DRD2 agonist, quinpirole, at the indicated concentrations versus control. One-way ANOVA for post-oral arm length, F 3,463 =30.586, P <0.0001. Bonferroni-corrected comparisons versus control; *** P <0.001. The decrease in arm length was not due to a global response or sick embryos as body rod length and other aspects of larval morphology did not change with treatment. ( b ) Change in post-oral arm and body rod length for 5-day larvae cultured with versus without algae for control (blue) and DRD2 antagonist amisulpride, 25 μM, (light grey) treatments. ANOVA ( Supplementary Table S1 ), treatment×algae for post-oral arms, F 1,363 =7.005, P =0.008 and for body rods, F 1,345 =1.584, P =0.209; Bonferroni-corrected comparisons without versus with algae (i.e. algae-induced change), *** P <0.001. Error bars±s.e.m. DRD2, dopamine receptor type-D 2 . Full size image For an independent test of involvement of the dopamine pathway in algal sensation, we disrupted tyrosine hydroxylase (TH) production and blocked TH activity to prevent dopamine biosynthesis ( Fig. 3 ; Supplementary Tables S2, S3 ). TH is required for the conversion of L -tyrosine to L-DOPA, the dopamine precursor, and is the rate-limiting enzyme in catecholamine biosynthesis. Microinjection of a translation-blocking morpholino antisense oligonucleotide (MASO) targeted to TH (TH MASO1), suppressed the post-oral arm response to algae ( Fig. 3a ). TH MASO1 morphants developed normally ( Fig. 3a ; Supplementary Fig. S1 ; Supplementary Table S2 ), but lacked detectable TH protein ( Fig. 3b ). A second TH morpholino ( Fig. 3c ) as well as pharmaceutical inhibition of TH withα-methyl-p-tyrosine ( Fig. 3d ) also suppressed the short-arm response to food, confirming the TH MASO1 morphant phenotype. 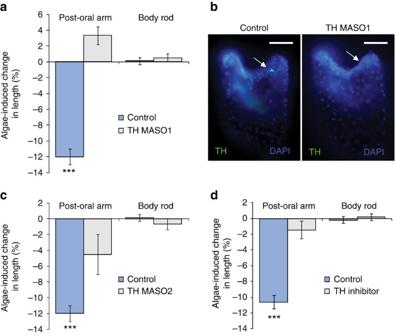Figure 3: Dopamine biosynthesis is necessary for the response to algae. (a) Change in post-oral arm and body rod length for 4-day larvae cultured with versus without algae for control (blue) and a translation-blocking MASO at 0.4 mM (TH MASO1, light grey) treatments. ANOVA (Supplementary Table S2), treatment×algae for post-oral arms,F1,286=19.604,P<0.001 and for body rods,F1,285=0.359,P=0.550. Bonferroni-corrected comparisons without versus with algae (i.e. algae-induced change), ***P<0.001. (b) TH protein was not detectible in TH MASO1-injected embryos 4 days pf (right panel,n=22/22 TH negative) as compared with controls (white arrow in left panel,n=3/26 TH negative). Nuclei stained with DAPI (blue). Scale bars, 50 μm. (c) Change in post-oral arm and body rod length for 4-day larvae cultured with versus without algae for control (blue) and a splice-blocking MASO at 0.15 mM (TH MASO2, light grey) treatments. Student's two-tailedt-test without versus with algae, ***P<0.001. (d) Change in post-oral arm and body rod length for 5-day larvae cultured with versus without algae in control (blue) and TH inhibitor (light grey) treatments. ANOVA (Supplementary Table S3), treatment×algae for post-oral arms,F1,300=13.708,P<0.001 and for body rods,F1,262=0.060,P=0.807. Bonferroni-corrected comparisons without versus with algae, ***P<0.001. Error bars±s.e.m. Figure 3: Dopamine biosynthesis is necessary for the response to algae. ( a ) Change in post-oral arm and body rod length for 4-day larvae cultured with versus without algae for control (blue) and a translation-blocking MASO at 0.4 mM (TH MASO1, light grey) treatments. ANOVA ( Supplementary Table S2 ), treatment×algae for post-oral arms, F 1,286 =19.604, P <0.001 and for body rods, F 1,285 =0.359, P =0.550. Bonferroni-corrected comparisons without versus with algae (i.e. algae-induced change), *** P <0.001. ( b ) TH protein was not detectible in TH MASO1-injected embryos 4 days pf (right panel, n =22/22 TH negative) as compared with controls (white arrow in left panel, n =3/26 TH negative). Nuclei stained with DAPI (blue). Scale bars, 50 μm. ( c ) Change in post-oral arm and body rod length for 4-day larvae cultured with versus without algae for control (blue) and a splice-blocking MASO at 0.15 mM (TH MASO2, light grey) treatments. Student's two-tailed t -test without versus with algae, *** P <0.001. ( d ) Change in post-oral arm and body rod length for 5-day larvae cultured with versus without algae in control (blue) and TH inhibitor (light grey) treatments. ANOVA ( Supplementary Table S3 ), treatment×algae for post-oral arms, F 1,300 =13.708, P <0.001 and for body rods, F 1,262 =0.060, P =0.807. Bonferroni-corrected comparisons without versus with algae, *** P <0.001. Error bars±s.e.m. Full size image The responses to pharmaceutical and gene knock-down perturbations of DRD2 and TH were specific, affecting the length of the post-oral arms, but not that of body rods, indicating a local response rather than a nonspecific, whole-embryo response ( Figs 2 and 3 ; Supplementary Fig. S1 ; Supplementary Tables S1-S3 ). These data suggest that dopamine signalling through a dopamine type-D 2 receptor is both sufficient to mimic the response to high algal concentrations and necessary to mediate it. Dopaminergic neurons develop in the tips of the post-oral arms at the appropriate time to mediate the short-arm response to algae. Cells expressing TH were first detected by immunostaining at the prism stage ( Fig. 4a,b ) at the onset of elongation of the post-oral arms ( Fig. 4c , black arrow), and persisted through embryonic skeletal elongation to the start of feeding ( Fig. 4d,e ). Dopamine, TH protein and dopa decarboxylase mRNA were each detected in cells near the post-oral arm tips of plutei, in close proximity to the overlying ectoderm and to the primary mesenchyme cells (PMCs) that fabricate the larval skeleton ( Fig. 4d-f ). TH-positive cells also express the neural marker, Synaptotagmin B [18] ( Supplementary Fig. S2 ), and extend processes along the length of the ciliary band ( Fig. 4e ), which could be involved in algal sensation. These data are consistent with the distribution of dopamine-positive cells in S. droebachiensis larvae [19] and a neurosensory function. Higher magnification (×40) of embryos double stained for dopamine and a PMC marker revealed that dopamine-positive cells were immediately adjacent to the PMCs ( Fig. 4g-j ). Although plastic phenotypic responses often involve neuro-stimulation of a secondary endocrine signal [9] , the close proximity of dopamine-positive cells to the PMCs and overlying ectoderm in the post-oral arms raises the possibility that dopamine may signal directly to one or both cell types to inhibit arm growth. 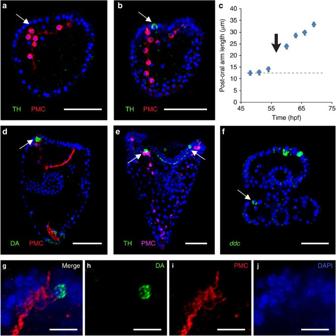Figure 4: Dopamine and dopamine biosynthesis enzymes are spatially and temporally expressed correctly to mediate the response to algae. Fluorescent immunohistochemical detection of the rate-limiting dopamine biosynthesis enzyme, TH, and a PMC marker (SM30) for reference, at 54 h post-fertilization (hpf) (a) and 60 hpf (b). White arrows in these and subsequent panels indicate the post-oral arm tip. (c) Post-oral arm length versus hpf showing coincident initiation of arm elongation and first detection of TH-positive cells (black arrow). Grey dashed line indicates approximate length of an initial triradiate spicule. Error bars±s.e.m. Fluorescent immunohistochemical detection of dopamine (d) and TH (e), and PMC markers, Msp130 (d) and SM30 (e), at pluteus stage (92 hpf). Fluorescent whole-mountin situhybridization detectingddcmRNA (f) in the post-oral arm tip and in the serotonergic ganglia (at the top of the image) at early pluteus (72 hpf, oral view). (g–j) Higher-magnification images of dopamine and PMC (Msp130) immunostains at the arm tip. Nuclei stained with DAPI (blue). DA, dopamineddc,dopa decarboxylase. Scale bars, (a–f) 50 μm, (g–j) 10 μm. Figure 4: Dopamine and dopamine biosynthesis enzymes are spatially and temporally expressed correctly to mediate the response to algae. Fluorescent immunohistochemical detection of the rate-limiting dopamine biosynthesis enzyme, TH, and a PMC marker (SM30) for reference, at 54 h post-fertilization (hpf) ( a ) and 60 hpf ( b ). White arrows in these and subsequent panels indicate the post-oral arm tip. ( c ) Post-oral arm length versus hpf showing coincident initiation of arm elongation and first detection of TH-positive cells (black arrow). Grey dashed line indicates approximate length of an initial triradiate spicule. Error bars±s.e.m. Fluorescent immunohistochemical detection of dopamine ( d ) and TH ( e ), and PMC markers, Msp130 ( d ) and SM30 ( e ), at pluteus stage (92 hpf). Fluorescent whole-mount in situ hybridization detecting ddc mRNA ( f ) in the post-oral arm tip and in the serotonergic ganglia (at the top of the image) at early pluteus (72 hpf, oral view). ( g–j ) Higher-magnification images of dopamine and PMC (Msp130) immunostains at the arm tip. Nuclei stained with DAPI (blue). DA, dopamine ddc , dopa decarboxylase . Scale bars, ( a–f ) 50 μm, ( g–j ) 10 μm. Full size image Gene knock-down ( Fig. 3 ) and pharmaceutical perturbation experiments ( Figs 2 and 3 ) targeting two independent points in the signalling pathway, together with the temporal and spatial expression patterns of dopamine and dopamine biosynthetic enzymes ( Fig. 4 ), identify dopamine as a key signal mediating the phenotypic response to food availability. In the absence of dopamine signalling, plasticity in arm length is lost. Thus the direction of the phenotypic plasticity is clear: short arms are induced at high food density when dopamine signalling inhibits skeletal elongation and thus feeding structure growth. Consequences for food acquisition and maternal lipid stores Showing the involvement of dopamine signalling established that the response is directed toward reducing the size of feeding arms and also allowed us to artificially manipulate the size of the feeding structure to determine the adaptive capacity. We tested the functional consequences for feeding and energy expenditure by pharmaceutically varying feeding apparatus size. This method was advantageous over varying algal concentrations because sea urchin larvae can incorporate exogenous dissolved organic material [20] , [21] that could change their metabolic state, even though they are not yet feeding. Previous studies have shown that the size of the feeding apparatus correlates well with the maximum food clearance rate over developmental time [13] , [22] and among different species [23] of echinoderm larvae. The differences in size are greater between species or development stages (for example, 4-arm versus 8-arm echinoplutei) than we have observed here at a single developmental stage in a single species. To determine whether the relatively small changes in feeding structure could significantly affect algal capture rates, we pharmaceutically manipulated feeding structure size and then allowed the larvae to feed on a suspension of algal mimics. Variation in post-oral arm length was significantly correlated with P <0.001 and explained ∼ 20% of the variation in bead ingestion rate at low densities (1,500 beads per ml; Fig. 5a ) and more than 25% of the variation at higher densities (4,000 beads per ml; Supplementary Fig. S3 ). The clearance rate increased 8.7% (±1.2% s.d.) at low densities food and 11.2% (±3.4% s.d.) at high food densities per 10% increase in post-oral arm length. Thus, differential arm elongation during the pre-feeding stage can alter individual fitness by varying the ciliary feeding capacity, and thus potential food intake rate. These, together with the dopamine perturbation results, lead to the conclusion that food induces a rapid morphogenetic response in pre-feeding sea urchin larvae that reduces food intake potential. 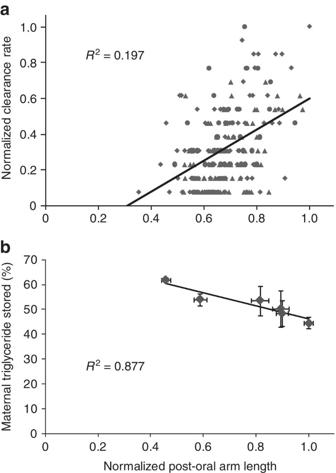Figure 5: Altering post-oral arm length confers a fitness advantage. (a) Regression of clearance rate on post-oral arm length at 5 days pf in replicate trials (circles, triangles and diamonds) at 1,500 beads per ml. Both variables were normalized relative to the observed maxima. Pooled Model I regression,R2=0.197, β1=0.866,P<0.001,n=203. (b) Regression of the mean percent of maternal triglyceride remaining on mean post-oral arm length, 5 days pf. The percent triglyceride was calculated as the amount of triglyceride on day 5 relative to the initial maternal triglyceride load in fertilized eggs, 0 day. Post-oral arm length was normalized to the maximum. Model II geometric mean regression,R2=0.877,β1=0.287±0.14 (95% CI),n=6. Error bars±s.e.m. Figure 5: Altering post-oral arm length confers a fitness advantage. ( a ) Regression of clearance rate on post-oral arm length at 5 days pf in replicate trials (circles, triangles and diamonds) at 1,500 beads per ml. Both variables were normalized relative to the observed maxima. Pooled Model I regression, R 2 =0.197, β 1 =0.866, P <0.001, n =203. ( b ) Regression of the mean percent of maternal triglyceride remaining on mean post-oral arm length, 5 days pf. The percent triglyceride was calculated as the amount of triglyceride on day 5 relative to the initial maternal triglyceride load in fertilized eggs, 0 day. Post-oral arm length was normalized to the maximum. Model II geometric mean regression, R 2 =0.877, β 1 =0.287±0.14 (95% CI), n =6. Error bars±s.e.m. Full size image The existence of a mechanism to suppress arm growth in high food densities despite the feeding advantage of longer arms seems counterintuitive and suggests that there must be a substantial cost to the long-armed phenotype of the pre-feeding larva. To test this idea, we next analysed the expenditure of maternal triglyceride stores over a range of pharmaceutically induced post-oral arm lengths. Triglycerides are the primary energetic lipids used during pre-feeding development to fuel construction of the feeding larva [24] , [25] . The amount of stored triglycerides, as a percentage of the initial maternal triglyceride investment, was significantly negatively correlated with post-oral arm length at the end of the pre-feeding stage, 5 days post fertilization (pf) ( Fig. 5b ). The larval culture with the shortest arms at 5 days pf had 62.0% (±0.7% s.e.m) of the initial triglycerides remaining compared with 44.6% (±2.2% s.e.m.) for the larval culture with the longest arms ( Fig. 5b ). Thus, embryos could variably conserve ∼ 15% of the maternal triglyceride load when dopamine signalling was strongly stimulated and larval arms were short. Assuming an average usage of ∼ 1 ng triglyceride per individual per day ( Supplementary Fig. S4 ), a savings of 15% represents more than 1 day of energy. This is a substantial cost early in larval life, as triglycerides are depleted by day 10 ( Supplementary Fig. S4 ) and are not replenished by feeding [25] . Developmental plasticity through dopamine signalling thus allows larvae to preserve a considerable proportion of maternal energetic reserves. The food response of sea urchin larvae, like many prey-induced traits, has been thought to be offensive and act to increase predator food acquisition [2] , [15] . In contrast, our data demonstrate that the molecular mechanism actually acts to reduce the size of the feeding structure when algae are detected. The algae-induced dopamine signalling suppresses the developmental 'default' programme operating in pre-feeding larvae to produce shorter arms with lower food acquisition potential. For phenotypic plasticity to be maintained, phenotypic changes should maximize fitness for the given environment. We show that the long-armed phenotype maximizes fitness when food is scarce through increased food acquisition potential at the expense of maternal lipids; whereas the short-armed phenotype maximizes fitness when food is abundant through conserving maternal lipids at the expense of maximum food acquisition potential. There may be additional fitness tradeoffs, for example between arm length and stomach size [26] and/or swimming performance [27] associated with this developmental response. Although the functional tradeoffs are bidirectional, the mechanism that establishes the phenotypes is a unidirectional response. Maximum food acquisition rates are the 'default' state constrained by the developmental programme and/or maternal inputs. Thus, increasing the size of the feeding apparatus beyond its current maximum, to compensate for potential decreases in food resources due to climate change, would require additional maternal investment and/or evolution of the developmental programme. The dopamine-signaling mechanism underlying the developmental plasticity is only induced when food is present, and increases in significance when food is abundant. Thus, natural selection has favored the existence of two programmes regulating larval arm growth: a developmental programme that optimizes food acquisition potential and another that confers developmental plasticity by adjusting the operation of this programme to, in part, optimize use of energy stores. An interpretation of this developmental response mechanism might be that there is a finite or diminishing return for increased ciliary feeding at high food concentrations, possibly due to physiological constraints [26] . However, benefits of the short-armed phenotype, which is induced by food through dopamine signalling, could be a driving factor whether or not ciliary feeding capacity (arm length) is limited. The ability to allocate maternal energy stores to other purposes could have substantial consequences for survival and performance success across multiple life-history stages through latent effects [28] , [29] , [30] . For example, through increased allocation towards development of the juvenile, larvae might be able to decrease the length of time they are exposed to predators in the plankton, or there might be an increase in the quality of the settled juveniles [29] , [30] . As S. purpuratus has a high post-settlement mortality rate with infrequent successful recruitment events [31] , [32] , condition at settlement could be an important factor controlling the dynamics of benthic sea urchin populations, which have community level consequences [33] , [34] . If mismatches between larval abundances and food availability increase in frequency or severity, the reduced algal abundances during the pre-feeding stage would result in an increased occurrence of long-armed larvae and a loss of any benefits of short-armed larvae, such as reallocation of maternal energy stores. Our data demonstrate the adaptive use of dopamine signalling to rapidly alter development of feeding structures in anticipation of food. Only by gaining a mechanistic understanding could this prey-induced change in form be placed in the appropriate ecological and also evolutionary context. Diverse organisms, from worms to humans, use dopamine signalling [35] , [36] , through dopamine type-D 2 receptors in particular [37] , [38] , to anticipate food consumption. However, in C. elegans [35] , [38] , insects [39] , [40] , adult sea urchins [41] , and mammals, including humans [36] , dopamine signalling alters behaviour in anticipation of food, whereas pre-feeding sea urchin larvae alter their development and form, as presented here. Thus, the dopamine signalling involved in regulating larval development may represent a co-option or redeployment of the highly conserved use of dopamine signalling in mediating behaviour in anticipation of food. Embryo and larval culture Adult sea urchins, Strongylocentrotus purpuratus , from Cultured Abalone and the Point Loma Marine Invertebrate Lab, CalTech were maintained in seawater at 10 °C. Gametes were harvested via intracoelomic injections of 0.55 M KCl. Embryos were cultured using standard methods at densities of 1–5 embryos per ml in artificial seawater (ASW) at 15 °C, with or without algae ( ∼ 5,000 cells per ml of Dunaliella sp.). Quantification of skeletal lengths Post-oral arm and body rod lengths ( n ≥20, each) were assayed from a random sample taken at 5 days pf, just before feeding begins, except for morpholino-injected embryos, which were sampled at 4 days pf to ensure that morpholino knockdown of TH protein synthesis was still effective. Larvae were squash mounted on microscope slides to position the skeletal elements in the same plane, and then imaged on a Zeiss Axiovert 200 M inverted microscope at ×20 under differential inference contrast, which readily identifies the birefringent skeletal elements. The skeletal lengths were quantified from the digital images using AxioVision software (Carl Zeiss MicroImaging). In some cases (<1%), a skeletal element could not be measured due to breakage or exit from the plane of focus. Pharmaceutical perturbations Dopamine signalling was perturbed using quinpirole, a widely used and specific type-D 2 receptor agonist [42] , amisulpride, a highly selective D 2 /D 3 dopamine receptor antagonist [43] , and α-Methyl-DL-tyrosine methyl ester hydrochloride, a selective inhibitor of TH [44] , administered directly via dilution into the culture medium (ASW) to full-sibling larvae at late gastrula stage (48–52 hpf), unless otherwise noted in the text. Pharmaceutical experiments were performed in duplicate with different female–male pairings. Microinjections Fertilized eggs were microinjected with filtered solutions containing 20% glycerol and rhodamine dextran without morpholinos (glycerol control), with 0.4 mM TH MASO1, or with 0.15 mM TH MASO2 using an Eppendorf Femtojet-Injectman NI2 micromanipulator attached to a Leica inverted fluorescent microscope, as in (ref. 45 ). TH MASO1 injections were replicated with two different female–male pairings. Glycerol and uninjected embryos were compared and no significant changes in skeletal lengths, TH immunostaining or response to algae were detected; thus, some later experiments used uninjected embryos as controls. The translation-blocking TH MASO1 was designed based on the predicted TH (GLEAN 00836) 5′UTR, which was confirmed by RACE. TH MASO1: 5′-GCGTCCTGCTGTAGAAGATACTTGA-3′. TH MASO2 targeted the intron 8/exon 9 boundary to disrupt the catalytic domain of the enzyme [46] . TH MASO2: 5′-GCCTACGATGAACAAGAACAAATGT-3′. Statistical analyses for dopamine perturbations The dose response of post-oral arm length to treatment with quinpirole was assessed using a one-way analysis of variance (ANOVA) and subsequent Bonferroni-corrected pair-wise comparisons versus the control to determine if the change relative to control was significant. The response to algae was assessed in pharmaceutical and TH MASO1 perturbations by a three-way ANOVA where perturbation treatment, algal treatment (with versus without algae) and experimental replicate were fixed effects and the mean square error was used as the denominator of the f-ratio [47] . Since all experiments showed a significant ( P >0.05) interaction between perturbation and algal treatments for post-oral arm length, subsequent Bonferroni-corrected pair-wise comparisons were performed to determine if the algae-induced change was significant. TH MASO2 was not replicated and was thus assessed using Student's two-tailed t -tests. All statistical analyses were done in SYSTAT v10 with output to three decimal places, thus exact P -values are given if P >0.001. Immunostains and fluorescence in situ hybridization Immunostains for dopamine (1:1500, ab6428, Abcam), TH (1:200, ImmunoStar), Msp130 (1:5, 6a9) [48] , SM30 (1:400, 3814, courtesy of F.H. Wilt) [49] and Synaptotagmin B (1:500, rat, courtesy of R. Burke) were performed as in (ref. 50 ). To determine the time of initial expression of TH, embryos were incubated in the TH antibody at 4 °C over two nights to improve sensitivity. Fluorescent whole-mount in situ hybridization for dopa decarboxylase was carried out as in (refs 45 , 51 ) except for inclusion of two more stringent post-hybridization washes in 70% hybridization buffer for 45 min each. Two fragments (470 and 758 bp) of the dopa decarboxylase gene isolated with primers: forward1, 5′-CTCCGATGATTTCCGTGTCT-3′; reverse1, 5′-CTGCCAGCAAGGCTACTAGA-3′; forward2, 5′-CCACCGATGACAAAGGTTCT-3′; and reverse2, 5′-CCAGGCATACGTCATGTGTC-3′ were used to generate probes used simultaneously to detect gene expression. Embryos were imaged using a Zeiss Axiovert 200 M inverted microscope at ×20 or ×40. Optical sections were obtained with an ApoTome unit (Zeiss) and stacked images were prepared using Imaris (Bitplane Inc.). Feeding experiment We treated half-sib larvae from three females with ASW (control), DRD2 agonist (quinpirole) and DRD2 antagonist (amisulpride) to maximize the size range of the feeding structures. Larvae from each of these treatments were combined into three replicate cultures, transferred to ASW for 4 h, and then allowed to feed on a gently stirred suspension of algal mimics, 10 μm Polybead Microspheres (Polysciences, Inc) coated with BSA at 1,500 or 4,000 beads per ml, for 45 min. The number of beads ingested and skeletal lengths were measured for at least 30 larvae from each replicate as above. There was no significant difference between replicate samples fed at 1,500 beads per ml (two-factor ANOVA, two-tailed P =0.950, SYSTAT v.10), so the replicates were pooled and analysed using a model I regression. Lipid analyses Duplicate cultures, each consisting of half-siblings from three females, were cultured in gently stirred 500 ml beakers within a 15 °C incubator. At the onset of arm elongation ( ∼ 65 hpf), the cultures were divided into three treatments: control, amisulpride 25 μM and quinpirole 50 μM. Replicate samples of 250 individuals each were collected from each treatment on days 0, 2, 3, 4, 5, 6, 8 and 10 pf and stored frozen at −80 °C until lipid analysis using an Iatroscan Mark 5 new TLC/FID (flame ionization detection). Lipid was extracted from frozen embryo and larval samples with ketone as an internal standard [24] . Immediately before spotting, the lipid extract was dried in a stream of N 2 gas and 10 μl of HPLC-grade chloroform was added using a Gilson positive displacement pipette. The rack containing 10 Chromarods was positioned on a warm hot plate during spotting of 5 μl of the lipid extract onto 8 individual Chromarods to ensure that the sample remained in a narrow band at the origin. The remaining two Chromarods were used to run an unspotted negative control [24] and a composite lipid standard to confirm peak identification and prepare standard curves for quantification of the 8 lipid classes [24] plus diglyceride. The Chromarods were run in a double development: hexane:diethyl ether:formic acid (98.5:1:0.05) for two sequential developments of 25 and 20 min followed by 5 min drying at 60 °C and a partial scan; 36 min in hexane:diethyl ether:formic acid (79:20:1), drying and a full scan. We present triglyceride concentrations for each treatment and time point based on lipid extracts obtained from three replicate samples, each containing 250 individuals, as a measurement of maternal energetic stores. Normalized, mean post-oral arm length and triglyceride levels were assessed using a Model II geometric mean regression [52] to take into account the error associated with both variables. Post-oral arm length was normalized to the maximum. Triglyceride concentration was normalized to the initial concentration in fertilized eggs (day 0, pre-cleavage). Treatments within a replicate culture had the same initial triglyceride concentrations, allowing for direct comparisons between treatments. As there was no interaction with cultures (two-factor ANOVA, two-tailed P =0.478, SYSTAT v.10), the two cultures were pooled for the regression. How to cite this article: Adams, D.K. et al . Rapid adaptation to food availability by a dopamine-mediated morphogenetic response. Nat. Commun. 2:592 doi: 10.1038/ncomms1603 (2011).